Extremotolerant tardigrade genome and improved radiotolerance of human cultured cells by tardigrade-unique protein Tardigrades, also known as water bears, are small aquatic animals. Some tardigrade species tolerate almost complete dehydration and exhibit extraordinary tolerance to various physical extremes in the dehydrated state. Here we determine a high-quality genome sequence of Ramazzottius varieornatus , one of the most stress-tolerant tardigrade species. Precise gene repertoire analyses reveal the presence of a small proportion (1.2% or less) of putative foreign genes, loss of gene pathways that promote stress damage, expansion of gene families related to ameliorating damage, and evolution and high expression of novel tardigrade-unique proteins. Minor changes in the gene expression profiles during dehydration and rehydration suggest constitutive expression of tolerance-related genes. Using human cultured cells, we demonstrate that a tardigrade-unique DNA-associating protein suppresses X-ray-induced DNA damage by ∼ 40% and improves radiotolerance. These findings indicate the relevance of tardigrade-unique proteins to tolerability and tardigrades could be a bountiful source of new protection genes and mechanisms. Tardigrades, also known as water bears, are tiny aquatic animals having four pairs of legs [1] . More than 1,000 species have been reported from various habitats such as marine, fresh water or limno-terrestrial environments. All tardigrades require surrounding water to grow and reproduce, but some species—typically those living in the limno-terrestrial environments—have the ability to tolerate almost complete dehydration. When encountering desiccation, tolerant tardigrades lose body water and enter a contracted dehydrated state called anhydrobiosis, which is a reversible ametabolic state. The dehydrated tardigrades withstand a wide range of physical extremes that normally disallow the survival of most organisms, such as extreme temperatures (from −273 °C [2] to nearly 100 °C [3] , [4] ), high pressure (7.5 GPa) [5] , immersion in organic solvent [4] , [6] , exposure to high dose of irradiation [7] , [8] and even direct exposure to open space [9] . Although such unusual tolerance of some tardigrades has long fascinated researchers, the molecular mechanisms enabling such exceptional tolerance have remained largely unknown. Recently, a finding was reported by a research group at the University of North Carolina (UNC) claiming the presence of extensive horizontal gene transfer (HGT) in a tardigrade genome (17.5% of genes have foreign origin) as a potential basis of tolerant ability, based on their own draft genome assembly of a freshwater tardigrade, Hypsibius dujardini (N50=15.9 kb; hereafter referred to as the UNC assembly) [10] . In contrast, another research group offered a counterargument, suggesting that a substantial portion of the UNC assembly were derived from contaminating microorganisms [11] . There is also a significant discrepancy between the estimated genome size of the species (80–110 Mbp) [11] and the span of the UNC assembly (212.3 Mb), which could be explained by the presence of contaminating sequences at least partially. It is controversial whether extensive HGT is real or an inaccurate interpretation of contaminating sequences. Contaminating sequences substantially affect genome analyses, leading to misinterpretation of the gene repertoire in the target organisms, as well as poor assembly or even chimeric misassembly. Metagenomic approaches could be used to identify putative contaminating sequences based on sequence similarity to phylogenetically distant taxa [11] , but possible misidentification and erroneous elimination from the assembly may lead to a biased representation of the gene repertoire for the target organism. A bona fide tardigrade genome sequence largely free from contamination is therefore needed. The possible contribution of foreign genes was discussed in the presumed tolerant ability of the sequenced species, H. dujardini [10] . However, freshwater tardigrades, including H. dujardini , are among the least tolerant members of the phylum Tardigrada and H. dujardini cannot withstand exposure to low humidity conditions without a long pre-exposure to high-humidity conditions [12] , [13] . Furthermore, no data have been reported for their tolerability against extreme stress in a dehydrated state, although they exhibit some tolerance to radiation in a hydrated state [14] . The controversial extensive HGT was thoroughly examined in the poorly tolerant H.dujardini , but no other gene repertoire analysis has been reported for tardigrades. Therefore, the genomic basis for the exceptional tolerance of tardigrades remains to be elucidated. To this end, we conducted a precise genome analysis using one of the most stress-tolerant tardigrade species, R. varieornatus , which tolerates direct exposure to low-humidity conditions and withstands various extremes in the dehydrated state [4] , [15] . We determined a high-quality genome sequence largely free from contamination that allows us to precisely analyse the gene repertoire, such as the proportion of HGT, and characteristic gene expansion or deletion. We also analysed the gene expression profiles during dehydration and rehydration. Furthermore, we focused on the abundantly expressed tardigrade-unique genes and present evidence for the relevance of tardigrade-unique proteins to tolerability, based on our investigation of the effect of a novel tardigrade-unique DNA-associating protein on DNA protection and radiotolerance in human cultured cells. High-quality genome sequence of extremotolerant tardigrade R. varieornatus is an extremotolerant tardigrade species, which becomes almost completely dehydrated on desiccation ( Fig. 1a,b ) and withstands various physical extremes [4] . 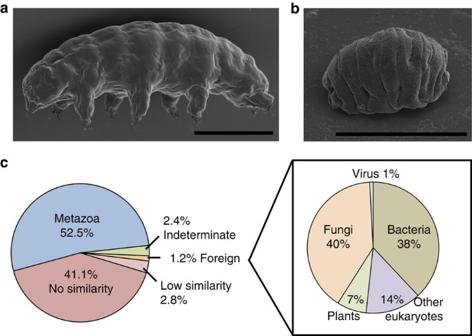Figure 1: The extremotolerant tardigradeR. varieornatusand taxonomic origins of its gene repertoire. (a,b) Scanning electron microscopy images of the extremotolerant tardigrade,R. varieornatus, in the hydrated condition (a) and in the dehydrated state (b), which is resistant to various physical extremes. Scale bars, 100 μm. (c) Classification of the gene repertoire ofR. varieornatus, according to their putative taxonomic origins and distribution of best-matched taxa in putative HGT genes. The genome sequence of R. varieornatus was determined by using a combination of the Sanger and Illumina technologies ( Supplementary Table 1 ). To minimize microbial contamination we cleansed egg surfaces with diluted hypochlorite and before sampling the tardigrades were starved and treated with antibiotics for 2 days. After the removal of short scaffolds (<1 kb) and mitochondrial sequences, we obtained the assembly spanning 56.0 Mbp (301 scaffolds). Coverage analysis (160 × Illumina sequencing) revealed that 199 scaffolds (99.7% in span) had considerable coverage (>40), whereas 102 scaffolds had exceptionally low coverage (<1; Supplementary Fig. 1 and Supplementary Data 1 ). We considered these 102 scaffolds (153 kb in span) as derived from contaminating organisms and excluded them from our assembly. 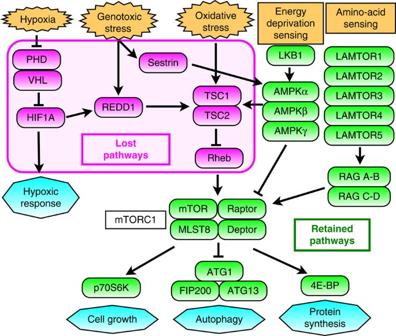Figure 2: Selective loss of stress responsive signalling to mTORC1 downregulation. Gene networks involved in the regulation of mTORC1 activity. Magenta indicates genes absent in the tardigrade genome and green indicates retained genes. The interconnected eight genes mediating environmental stress stimuli to downregulate mTORC1 were selectively lost, whereas all components involved in sensing and mediating physiologic demands were present. As a result, our final assembly spans 55.8 Mbp (199 scaffolds; N50=4.74 Mbp; N90=1.3 Mbp; Supplementary Table 2 ). The span is highly concordant with the genome size estimated by DNA staining in the tardigrade cells ( ∼ 55 Mbp; Supplementary Fig. 2 ), suggesting sufficiency of our assembly span and no significant inflation by contaminated organisms. We also constructed a full-length complementary DNA library from dehydrated tardigrades and determined paired-end sequences. BLAST search of these Expression Sequence Tag (EST) data against our genome assembly revealed 70,674 of 70,819 sequences (99.8%) were successfully mapped ( E -value<10 65 ). The completeness of our assembly was also supported by high coverage (95.6%) in essential eukaryotic genes assessed by Core Eukaryotic Genes Mapping Approach [16] ( Supplementary Table 2 ) and the very low duplication rate in Core Eukaryotic Genes Mapping Approach (1.13) indicated that our assembly was largely free from inflation by contaminating organisms. We generated gene models based on our messenger RNA-sequencing (RNA-seq) data for six states (two embryonic stages and four states of adults during dehydration and rehydration) and merged them with ab initio gene models, to produce the comprehensive gene set, containing 19,521 protein-coding genes. 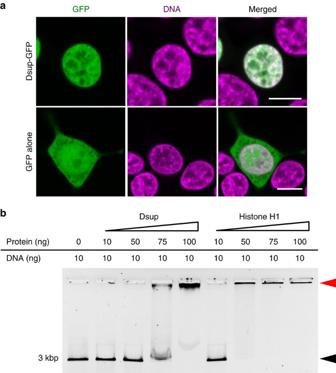Figure 3: Co-localization with nuclear DNA and mobility shift of DNA by Dsup. (a) Subcellular localization of Dsup-GFP fusion proteins transiently expressed in HEK293T cells. Nuclear DNA was visualized by Hoechst 33342. Scale bars, 10 μm. (b) Mobility shift of DNA by bacterially expressed Dsup protein in a dose-dependent manner (10, 50, 75 or 100 ng). Black arrowhead indicates the predicted size of the probe DNA (3 kbp, 10 ng). Red arrowhead indicates the position of the extremely slowly migrating DNA in the presence of Dsup protein. A similar extensive mobility shift was observed with histone H1. The genome of this species was highly compact and, correspondingly, the mean length of coding sequences (1,062 bp), exons (234 bp) and introns (402 bp) were fairly short and genes were densely distributed with short inter-coding sequence distances (mean 1,099 bp; Supplementary Table 3 ). Figure 1: The extremotolerant tardigrade R. varieornatus and taxonomic origins of its gene repertoire. ( a , b ) Scanning electron microscopy images of the extremotolerant tardigrade, R. varieornatus , in the hydrated condition ( a ) and in the dehydrated state ( b ), which is resistant to various physical extremes. Scale bars, 100 μm. ( c ) Classification of the gene repertoire of R. varieornatus , according to their putative taxonomic origins and distribution of best-matched taxa in putative HGT genes. Full size image No extensive HGT in R. varieornatus genome To evaluate the significance of HGT in the tardigrade gene repertoire, we first performed BLAST search against the non-redundant database of National Centre for Biotechnology Information. Among the 19,521 tardigrade proteins, 10,957 proteins (56.1%) had similar proteins below the threshold ( E -value≤10 −5 ) used to estimate HGT in rotifers [17] . The vast majority exhibited the best similarity with metazoan proteins and were thus classified as metazoan origin (10,249 proteins; 52.5% of total proteins; Fig. 1c ). We examined putative HGT based on HGT indices that were calculated by subtracting the best bit score of the metazoan hit from that of the non-metazoan hit in BLAST searches, as used in previous reports [10] , [17] . Only 234 proteins (1.2%) had HGT scores higher than the previously defined threshold (≥30) [10] , [17] and were classified as putative HGT genes ( Fig. 1c and Supplementary Data 2 ). Of 234 putative HGT genes, 226 genes were encoded in the scaffolds containing metazoan-origin genes and all 234 putative HGT genes were supported by substantial coverage of genomic reads ( Supplementary Fig. 3 and Supplementary Data 2 ), suggesting that these putative HGT genes were encoded in the tardigrade genome rather than mis-incorporated minor contaminating sequences. In our evaluation of genome assembly, we excluded 102 scaffolds due to the extremely low coverage as a sign of possible contamination origins. To examine the impact of this exclusion on the estimated HGT proportion, we applied the same gene prediction on the excluded scaffolds and found 152 additional protein-coding genes. Of these 152 genes, 129 exhibited high HGT indices (≥30) and were classified as putative HGT genes. Even taking into account these genes, the proportion of putative HGT genes was still only 1.8% ( Supplementary Table 2 ). In any case, the proportion of HGT in our genome was much lower than those reported for the UNC assembly of H. dujardini (17.5%) [10] . In addition to the HGT proportion, we also found a striking contrast in putative taxonomic origins of HGT genes. In the UNC assembly, most (>90%) of the putative HGT genes were presumed to be of bacterial origin. In contrast, more than half (65%) of the putative HGT genes have probable eukaryotic origins in our assembly, mainly fungal origin ( Fig. 1c ). Our transcriptome analyses revealed that 138 of 234 putative HGT genes were certainly transcribed (fragments per kilobase of exon per million mapped fragments ≥5) and were considered as functional ( Supplementary Data 2 ). These functional HGT genes included several tolerance-related genes, for example, catalases. Catalase is an antioxidant enzyme that decomposes hydrogen peroxide, which is hazardous to the organism, and antioxidant enzymes are presumed important to counteract oxidative stress during desiccation [18] . In our assembly, we found three catalases and one putative pseudo-gene. All of them had high HGT scores and contained an extra domain at the carboxy terminus compared with other metazoan catalases ( Supplementary Fig. 4 ). This structure resembles those of bacterial clade II catalases. Catalases are classified into three sub-groups, termed clade I, II and III, and all other metazoan catalases are classified as clade III [19] . Phylogenetic analyses confirmed the classification of tardigrade catalases as clade II ( Supplementary Fig. 5 ). Expansion of stress-related genes in the tardigrade genome Comparison of the gene repertoire with other metazoans revealed characteristic expansion of several stress-related gene families such as superoxide dismutases (SODs) and MRE11 ( Supplementary Fig. 6 and Supplementary Data 3 ). Sixteen SODs were found in our assembly, whereas less than ten SODs are found in most metazoans. SOD is a detoxifying enzyme of superoxide radicals, a type of reactive oxygen species (ROS) [18] . As desiccation induces oxidative stress, expanded SODs could contribute to better tolerance against desiccation [18] . MRE11, another expanded gene family, plays important roles in repair processes of DNA double-strand breaks (DSBs) [20] . Four MRE11 genes were found in our assembly, whereas most animals possess only one copy. DNA in tardigrade cells undergo DSBs during long preservation in a dehydrated state and expanded MRE11 might be beneficial for efficient repairing damaged DNA. In the UNC assembly of H. dujardini , expansions by HGT were reported for several other DNA repair genes such as Ku , umuC , Ada and recA ( Rad51 ) [10] . We observed no significant expansion or sign of HGT for those genes in R. varieornatus ( Supplementary Data 3 ). Furthermore, all MRE11 genes in R. varieornatus were suggested to be of metazoan origin ( Supplementary Data 2 ). Thus, the expansion of MRE11 was likely to be due to gene duplication events during evolution to this lineage, rather than acquisition from other non-metazoan organisms through HGT. We also detected the expansion of some other gene families, for example, guanylate cyclases ( Supplementary Fig. 6 ). Their relation to tardigrade physiology is, however, currently elusive. Selective loss of peroxisomal oxidative pathway We also evaluated whether some metabolic pathways had been lost in our tardigrade genome. To assess this, we mapped genes found in model organisms but missing in our tardigrade genome to Kyoto Encyclopedia of Genes and Genomes (KEGG) pathways [21] . Statistical analysis revealed the significant gene loss in the peroxisomal pathway (corrected P -value=0.007, Fisher’s exact test; Supplementary Data 4 ). Many oxidative enzymes including those in the conserved β-oxidation pathway and several peroxisome biogenesis factors were missing ( Supplementary Figs 7 and 8 ). β-Oxidation is a major catabolic pathway of fatty acids, normally catalysed by two sets of enzymes, one in the mitochondria and the other in the peroxisome [22] . All members of the peroxisomal set were missing, whereas a complete set of mitochondrial enzymes was present ( Supplementary Data 5 ), suggesting actual gene loss in the peroxisomal β-oxidation process rather than insufficient genome sequencing. Selective loss of stress responsive pathways In addition to the KEGG pathways, we searched for the non-curated gene networks lost in the tardigrade genome by connecting putative lost genes using the protein–protein interaction database, STRING [23] . We found that eight lost genes had an interconnected network in the highly conserved stress-responsive signalling pathways ( Fig. 2 and Supplementary Data 6 ). Three of these genes, HIF1A , PHD and VHL , are central components to regulate response to hypoxia [24] . REDD1 is a downstream target of HIF1A [25] , as well as a downstream target induced by p53 on genotoxic stress [26] . REDD1 activates the TSC1/TSC2 complex, leading to downregulation of mammalian target of rapamycin complex 1 (mTORC1) activity [25] . The other lost gene, Sestrin , is also a downstream gene of p53 connecting genotoxic stress to mTOR signalling [27] . As TSC1/TSC2 is activated by oxidative stress [28] , the tardigrade lacks the signalling components connecting various stresses such as hypoxia, genotoxic stress and oxidative stress, to downregulation of mTORC1. In contrast, all other signalling components are present for regulation of mTORC1, depending on physiologic demands such as energy deprivation sensing [29] and amino acid sensing [30] . Figure 2: Selective loss of stress responsive signalling to mTORC1 downregulation. Gene networks involved in the regulation of mTORC1 activity. Magenta indicates genes absent in the tardigrade genome and green indicates retained genes. The interconnected eight genes mediating environmental stress stimuli to downregulate mTORC1 were selectively lost, whereas all components involved in sensing and mediating physiologic demands were present. Full size image Constitutive abundant expression of tardigrade-unique genes We examined gene expression profiles during dehydration and rehydration using mRNA sequencing and comparative analyses detected only minor differences ( Supplementary Data 2 ), suggesting that the tardigrade can enter a dehydrated state without significant transcriptional regulation. This finding is consistent with the fact that this tardigrade, R. varieornatus , tolerates rapid desiccation by direct exposure to low humidity conditions. We speculated that putative protective proteins are constitutively expressed. During inspection of abundantly expressed genes, we noticed that many abundantly expressed genes are classified as tardigrade-unique genes that exhibited no or low similarity to non-tardigrade proteins ( Supplementary Fig. 9 ). These abundantly expressed proteins included previously identified tardigrade-unique heat-soluble proteins, CAHS and SAHS, both of which maintain solubility even after heat treatment and are proposed to be involved in the protection of biomolecules during desiccation [31] , [32] . We found significant expansion of these tardigrade-unique protein families, as 16 CAHS genes and 13 SAHS genes in our assembly, whereas no counterparts were found in other phyla, except 3 SAHS genes with low similarity to several metazoan fatty acid-binding proteins. In accordance with the identification of CAHS and SAHS proteins as predominant proteins in the heat-soluble proteome of the tardigrade, our transcriptome data confirmed the abundant expression of these family members in the adult stage as well as in embryonic stages, although dominantly expressed members differed depending on the stage ( Supplementary Data 2 ). We found a reasonable number of genes unique to the species or the phylum (8,023 genes; 41.1% of the gene repertoire; Fig. 1c ). Abundantly expressed unique genes might be good candidates involved in the tolerability of the tardigrade. Identification of a tardigrade-unique DNA-associated protein R. varieornatus exhibits extraordinary tolerance against high-dose radiation [4] . Considering DNA as a major target of radiation damage, we hypothesized that tardigrade-unique proteins associate with DNA to protect and/or to effectively repair DNA in the tardigrade. To explore this possibility, we isolated the chromatin fraction from the tardigrade and used tandem mass spectrometry to identify the proteins contained in the bands selective to the chromatin fraction ( Supplementary Fig. 10 ). Among the identified proteins ( Supplementary Tables 4 and 5 ), we examined subcellular localization of putative nuclear proteins by expressing them as green fluorescent protein (GFP)-fused proteins in Drosophila Schneider 2 (S2) cells. Only one protein, termed Damage suppressor (Dsup), co-localized with nuclear DNA ( Supplementary Fig. 11 ) and similar co-localization was also observed in human cultured HEK 293T cells ( Fig. 3a ). Our transcriptome data revealed abundant expression of Dsup in an early embryonic stage (within the top 100 abundantly expressed genes; Supplementary Data 2 ), which is consistent because nuclear DNA extensively replicates in the embryonic stage. To verify the localization of Dsup protein in tardigrade cells, we performed immunohistochemistry with frozen sections of tardigrade embryos. In almost all tardigrade cells expressing Dsup, Dsup proteins co-localized with nuclear DNA ( Supplementary Fig. 12 ). Figure 3: Co-localization with nuclear DNA and mobility shift of DNA by Dsup. ( a ) Subcellular localization of Dsup-GFP fusion proteins transiently expressed in HEK293T cells. Nuclear DNA was visualized by Hoechst 33342. Scale bars, 10 μm. ( b ) Mobility shift of DNA by bacterially expressed Dsup protein in a dose-dependent manner (10, 50, 75 or 100 ng). Black arrowhead indicates the predicted size of the probe DNA (3 kbp, 10 ng). Red arrowhead indicates the position of the extremely slowly migrating DNA in the presence of Dsup protein. A similar extensive mobility shift was observed with histone H1. Full size image Dsup protein showed no sequence similarity to any proteins or motifs in BLASTP and InterProScan searches. In silico prediction revealed a putative long α-helical region in the middle and a putative nuclear localization signal at the C terminus ( Supplementary Fig. 13 ). Dsup protein is highly basic (pI=10.55), especially in the C-terminal region, suggesting its potential association with DNA through electrostatic interactions. Mutational analyses using variously truncated Dsup proteins fused with GFP revealed that the C-terminal region (Dsup-C) is required and sufficient for co-localization with nuclear DNA ( Supplementary Fig. 14a–c ). Expression of Dsup-C induced an abnormally aggregated distribution of nuclear DNA, whereas full-length Dsup-expressing cells had an almost normal distribution of nuclear DNA, similar to that in control cells ( Supplementary Figs 14a and 15 ). To examine the affinity of Dsup protein to DNA, we performed a gel-shift assay using bacterially expressed Dsup protein in vitro . Pre-incubation with purified Dsup protein significantly retarded the migration of linearized plasmid DNA in a dose-dependent manner ( Fig. 3b ), suggesting that Dsup protein has certain affinity to DNA in vitro . When Dsup protein was mixed with DNA at a 10:1 (wt:wt) ratio, the migration of DNA was almost completely inhibited. This retarded mobility of DNA could be due to formation of huge DNA–Dsup protein complexes and/or neutralization of the negative charge of DNA. These results suggested the physical affinity of Dsup protein to DNA molecules, although physiological specificity and mode of interaction between Dsup protein and DNA remain elusive. A similar drastic band shift was observed with the ubiquitous chromatin protein histone H1 (ref. 33 ). Dsup protein required the higher protein:DNA ratio for a complete band shift compared with histone H1, suggesting relatively weak affinity to DNA of Dsup than histone H1. Dsup protein lacking the C-terminal region (DsupΔC) completely lost the ability to shift the DNA mobility and Dsup-C alone was sufficient to shift the DNA band ( Supplementary Fig. 14d ). These findings indicated that the C-terminal region of Dsup is responsible for association with DNA as well as for co-localization with nuclear DNA. Dsup protein suppresses DNA damage in human cultured cells We hypothesized that the association of Dsup proteins with nuclear DNA might help to protect DNA from irradiation stress. To examine this possibility, we established a HEK293 cell line stably expressing Dsup under the control of the constitutive CAG promoter. Co-localization of Dsup protein with nuclear DNA was confirmed by immunocytochemistry in the established line ( Supplementary Fig. 16a ). X-ray irradiation induces various types of DNA damage, including DNA breaks, mainly single-strand breaks (SSBs). To examine the effect of Dsup on X-ray-induced DNA breaks, Dsup-expressing cells and untransfected HEK293 cells were exposed to 10 Gy X-ray irradiation. After irradiation, the cells were exposed to an alkaline condition (pH>13) to denature the damaged DNA and dissociated single-strand DNA fragments were analysed in single-cell electrophoresis (alkaline comet assay). The short fragmented DNA migrated to more distant location from the nuclei (comet tail region) and thus the proportion of DNA in the comet tail was considered an indicator of DNA breaks. In irradiated Dsup-expressing cells, the proportion of tail DNA was only 16%—less than half of that in the untransfected HEK293 cells (33%; Fig. 4a ). This finding suggested that Dsup protein suppressed X-ray-induced SSBs in human cultured cells. There are two modes for X-ray to induce SSBs: the direct absorption of X-ray energy into the DNA (direct effects) and through attack by ROS generated from water molecules activated by X-ray energy (indirect effects) [34] . We, therefore, examined the effect of Dsup protein on DNA SSBs generation by ROS. Exposure to hydrogen peroxide induced severe fragmentation of DNA (71% of total DNA in tail) in control HEK293 cells. In contrast, DNA fragmentation in Dsup-expressing cells was substantially suppressed to only 18% of total DNA in the tail ( Fig. 4b ), indicating that Dsup protein was able to protect DNA from ROS as well as X-rays. Pretreatment with the antioxidant, N -acetyl- L -cysteine (NAC) also substantially suppressed peroxide-induced SSBs. The combination of NAC and Dsup led to even greater suppression, although the suppression induced by their combination was less than the sum of those in each condition individually, suggesting that NAC and Dsup at least partially share the same suppression mechanism, most probably counteracting oxidative stress. 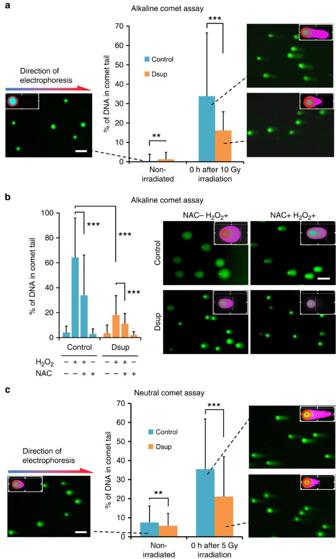Figure 4: Dsup protein suppresses stress-induced DNA fragmentation in human cultured cells. (a) The effects of Dsup on SSBs by 10 Gy X-ray irradiation in alkaline comet assays. The irradiated cells were immediately subjected to the assay. Representative images are shown for each condition. In the pseudo-coloured images in the inset, red to blue circles indicate nuclear DNA and magenta indicates fragmented DNA in tail. DNA fragmentation was assessed by the proportion of DNA detected in the tail region (% of DNA in Comet Tail). At least 281 comets were analysed for each condition. **P<0.01 and ***P<0.001 (Welch’st-test: non-irradiated,t-value=−3.199,P-value=0.0015; irradiated:t-value=8.599,P-value<1.0E−15). (b) The effects of Dsup on SSBs caused by hydrogen peroxide (H2O2) treatment in alkaline comet assays. Cells were treated with 100 μM H2O2for 30 min at 4 °C, to induce DNA damage with or without pretreatment with 10 mM NAC as an antioxidant for 30 min. At least 203 comets were analysed for each condition. ***P<0.001 (Tukey–Kramer’s test). (c) The effects of Dsup on DSBs by 5 Gy X-ray irradiation in neutral comet assays. Three hundred comets were analysed for each condition. **P<0.01 and ***P<0.001 (Welch’st-test: non-irradiated,t-value=2.758,P-value=0.0060; irradiated;t-value=7.406,P-value=4.7E−13). Values represent mean±s.d. in all panels. Scale bars, 100 μm. Figure 4: Dsup protein suppresses stress-induced DNA fragmentation in human cultured cells. ( a ) The effects of Dsup on SSBs by 10 Gy X-ray irradiation in alkaline comet assays. The irradiated cells were immediately subjected to the assay. Representative images are shown for each condition. In the pseudo-coloured images in the inset, red to blue circles indicate nuclear DNA and magenta indicates fragmented DNA in tail. DNA fragmentation was assessed by the proportion of DNA detected in the tail region (% of DNA in Comet Tail). At least 281 comets were analysed for each condition. ** P <0.01 and *** P <0.001 (Welch’s t -test: non-irradiated, t -value=−3.199, P -value=0.0015; irradiated: t -value=8.599, P -value<1.0 E −15). ( b ) The effects of Dsup on SSBs caused by hydrogen peroxide (H 2 O 2 ) treatment in alkaline comet assays. Cells were treated with 100 μM H 2 O 2 for 30 min at 4 °C, to induce DNA damage with or without pretreatment with 10 mM NAC as an antioxidant for 30 min. At least 203 comets were analysed for each condition. *** P <0.001 (Tukey–Kramer’s test). ( c ) The effects of Dsup on DSBs by 5 Gy X-ray irradiation in neutral comet assays. Three hundred comets were analysed for each condition. ** P <0.01 and *** P <0.001 (Welch’s t -test: non-irradiated, t -value=2.758, P -value=0.0060; irradiated; t -value=7.406, P -value=4.7 E −13). Values represent mean±s.d. in all panels. Scale bars, 100 μm. Full size image Besides SSBs, high-dose X-ray irradiation also induces DSBs, which are much more hazardous for organisms due to their difficult repair. We next examined the effect of Dsup protein on DSBs using a neutral comet assay, in which DNA fragmentation was analysed without dissociating in a neutral condition. The proportion of fragmented DNA was ∼ 40% reduced in Dsup-expressing cells compared with that in the untransfected cells ( Fig. 4c ). These findings together suggest that Dsup protein suppressed X-ray-induced DNA DSBs and SSBs. We further verified the suppression of DNA breaks by Dsup proteins using another DSB quantification method. In irradiated cells, histone H2AX around DSBs becomes phosphorylated within an hour [35] , referred to as γ-H2AX, and γ-H2AX can be used as an indicator of DSBs. We visualized γ-H2AX by immunofluorescence and counted the number of foci per nucleus at 1 h after irradiation. For this experiment, we irradiated cells with a relatively lower dose (1 Gy) of X-ray to avoid overlap of neighbouring foci and minimize counting errors. The Dsup-expressing cells exhibited an ∼ 40% reduced number of γ-H2AX foci compared with untransfected cells ( Fig. 5a ). We further established Dsup knockdown cells by transfecting a small hairpin RNA (shRNA) expression construct in Dsup-expressing cells. Dsup expression was successfully reduced by 77% in the knockdown cells ( Fig. 5b ). The reduction of DNA damage completely disappeared by Dsup knockdown ( Fig. 5c,d ). These findings indicated that Dsup protein is responsible for suppressing DNA damage in irradiated human cultured cells. When using a stable line expressing mutant Dsup protein, DsupΔC, which lacks the C-terminal DNA-associating region ( Supplementary Fig. 16b ), we detected no reduction of DNA fragmentation in the alkaline comet assays ( Supplementary Fig. 17a ), suggesting that the association with DNA is prerequisite for Dsup protein to protect DNA from X-ray. This view was further supported by the impaired suppression of the γ-H2AX foci in the DsupΔC-expressing cells ( Supplementary Fig. 17b ). 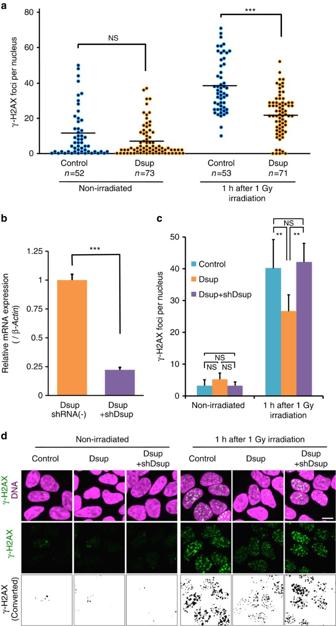Figure 5: Reduced formation of γ-H2AX foci in human cultured cells depending on Dsup expression. (a) Distribution of the numbers of γ-H2AX foci per nucleus is shown. Each dot represents an individual nucleus of a HEK293 cell (Control) or a Dsup-expressing cell (Dsup) under non-irradiated and irradiated conditions. ***P<0.001; NS, not significant (Welch’st-test). (b) Significant decrease ofDsuptranscript in shRNA-introduced cells (Dsup+shDsup) compared with that in untreated Dsup-expressing cells (Dsup shRNA(−)).n=3. Values represent mean±s.e.m. ***P<0.001 (Student’st-test). (c) Quantitative comparison of γ-H2AX foci number among untransfected HEK293 cells (Control), Dsup-expressing cells (Dsup) and Dsup-knockdown cells (Dsup+shDsup) under non-irradiated and 1 Gy X-ray irradiated conditions. At least 70 cells were analysed for each condition. Values represent mean±s.d. **P<0.01; NS indicates not significant (Tukey–Kramer’s test). (d) Representative images detecting γ-H2AX foci in each condition. Fluorescent images were converted to binary images for automatic counting of foci. Scale bar, 10 μm. Figure 5: Reduced formation of γ-H2AX foci in human cultured cells depending on Dsup expression. ( a ) Distribution of the numbers of γ-H2AX foci per nucleus is shown. Each dot represents an individual nucleus of a HEK293 cell (Control) or a Dsup-expressing cell (Dsup) under non-irradiated and irradiated conditions. *** P <0.001; NS, not significant (Welch’s t -test). ( b ) Significant decrease of Dsup transcript in shRNA-introduced cells (Dsup+shDsup) compared with that in untreated Dsup-expressing cells (Dsup shRNA(−)). n =3. Values represent mean±s.e.m. *** P <0.001 (Student’s t -test). ( c ) Quantitative comparison of γ-H2AX foci number among untransfected HEK293 cells (Control), Dsup-expressing cells (Dsup) and Dsup-knockdown cells (Dsup+shDsup) under non-irradiated and 1 Gy X-ray irradiated conditions. At least 70 cells were analysed for each condition. Values represent mean±s.d. ** P <0.01; NS indicates not significant (Tukey–Kramer’s test). ( d ) Representative images detecting γ-H2AX foci in each condition. Fluorescent images were converted to binary images for automatic counting of foci. Scale bar, 10 μm. Full size image Dsup improves viability of irradiated human cultured cells To test whether DNA protection by Dsup protein could also improve cellular survival after irradiation, we measured the cell viability after irradiation. In general, 3–7 Gy of X-ray induces severe DNA damage in mammalian cells, leading to loss of proliferative ability [36] . Accordingly, we irradiated cells with 4 Gy X-ray at 1 day post seeding (dps), which was the minimum dose enough to suppress proliferation of untransfected HEK293 cells in our condition. After irradiation, cell proliferation was examined at 24 h intervals for 8 days using PrestoBlue Cell Viability reagent, which measures the total reducing power of the cell culture [37] . Dsup-expressing cells exhibited slightly better cell viability after irradiation compared with those of untransfected HEK293 cells ( Supplementary Fig. 18a–c ). At 4 days after the cell viability analysis (12 dps), we noticed a drastic difference between Dsup-expressing cells and untransfected cells under phase-contrast microscopy ( Supplementary Fig. 18d ). Almost all irradiated untransfected cells had an abnormal round shape and were mostly detached from the culture dish, typical characteristics of dead cells. In contrast, many irradiated Dsup-expressing cells had a normal morphology and attached to the culture dishes, suggesting that these cells retained the characteristics of live adherent cells and perhaps even had proliferative ability. To confirm their proliferative ability, we examined the temporal change in cell numbers over a longer period after irradiation with 4 Gy of X-ray. Even under non-irradiated conditions, Dsup-expressing cells proliferated slightly faster than the untransfected cells, whereas Dsup-knockdown cells exhibited similar proliferation to that of untransfected cells ( Fig. 6b ). At 10–12 dps, the cell numbers became nearly saturated. Under irradiated conditions, almost all untransfected cells detached from the culture dish and had an abnormal round shape ( Fig. 6a ). In contrast, some of the irradiated Dsup-expressing cells attached to the culture dish with an apparently normal morphology and such cells increased over time ( Fig. 6a ). Cell counting analyses confirmed these observations. At 8 dps, the number of irradiated untransfected cells was almost unchanged from that at the seeding and further decreased at 10 and 12 dps ( Fig. 6b ). In contrast, the number of Dsup-expressing cells increased even at 8 dps compared with that at the seeding and drastically increased at 10 and 12 dps ( Fig. 6b ), suggesting that at least some fraction of irradiated Dsup-expressing cells retained proliferative ability. Growth rates at 8–12 dps were comparable to those of non-irradiated Dsup-expressing cells. In Dsup-knockdown cells, the improvements in cell viability and proliferative ability were completely abolished and their phenotypes were similar to those of untransfected HEK293 cells ( Fig. 6 ). These findings suggested that Dsup protein confers increased radiotolerance to human cultured cells. Cells expressing a Dsup mutant lacking the DNA-associating domain (DsupΔC) exhibited impaired improvement of radiotolerance compared with those expressing full-length Dsup protein ( Supplementary Fig. 19 ), suggesting that DNA targeting is important for full improvement of the radiotolerance by Dsup. As radiosensitivity of mammalian cells is affected by the cell cycle [38] , we compared the cell cycle distribution between Dsup-expressing cells and untransfected cells using flow cytometry. However, no significant differences were detected ( Supplementary Fig. 20 ), suggesting that the improved radiotolerance conferred by Dsup protein was not due to alterations of the cell cycle. 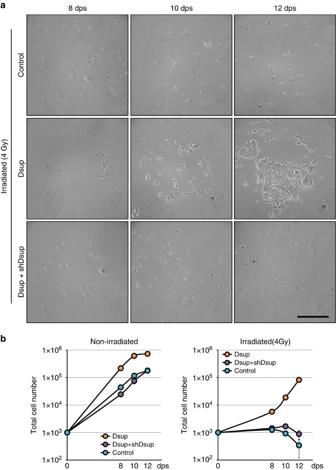Figure 6: Improved viability and proliferative ability of Dsup-expressing cells after irradiation. (a) Representative microscopic images with phase contrast at 8, 10 and 12 dps, of untransfected HEK293 cells (Control), Dsup-expressing cells (Dsup) andDsup-knockdown cells (Dsup+shDsup) irradiated with 4 Gy X-ray at 1 dps. Scale bar, 200 μm. (b) Comparison of growth curves of untransfected cells (Control), Dsup-expressing cells (Dsup) and Dsup-knockdown cells (Dsup+shDsup) in non-irradiated and irradiated conditions. Values represent mean±s.d. Figure 6: Improved viability and proliferative ability of Dsup-expressing cells after irradiation. ( a ) Representative microscopic images with phase contrast at 8, 10 and 12 dps, of untransfected HEK293 cells (Control), Dsup-expressing cells (Dsup) and Dsup -knockdown cells (Dsup+shDsup) irradiated with 4 Gy X-ray at 1 dps. Scale bar, 200 μm. ( b ) Comparison of growth curves of untransfected cells (Control), Dsup-expressing cells (Dsup) and Dsup-knockdown cells (Dsup+shDsup) in non-irradiated and irradiated conditions. Values represent mean±s.d. Full size image The genome sequence of R. varieornatus determined in this study is the first example of an extremotolerant tardigrade genome. All examined data, including congruence of the assembly span with the estimated genome size, and high coverage of EST and a core eukaryotic gene set, support the completeness of the determined genome sequence. The clear separation of minor contaminating scaffolds based on coverage and the consistent GC proportion and coverage of the scaffolds in the final assembly suggested that our assembly is largely free from contamination. The quality of our assembly is two orders of magnitude better (N50 ∼ 4.7 Mb) than those of the two draft genomes of the freshwater tardigrade, H. dujardini (N50 ∼ 15.9 or 50.5 kb) and thus could be useful as a reference genome of the phylum. The estimated HGT proportion (1.2%) in our final assembly is one order of magnitude lower than that in the controversial UNC assembly of H. dujardini (17.5% HGT) [10] . We did not exclude any sequences from the assembly based on sequence similarity to foreign organisms (for example, bacteria) and thus there was no preferential removal of HGT genes and no bias to underestimate the HGT proportion. The HGT index is a useful indicator for the possibility of HGT, but is not a sufficient criterion to guarantee true HGT. Indeed, previous phylogenetic analyses validated only an average of 55% of the genes with a high HGT index (≥30) as foreign origin [39] . Thus, our estimated HGT proportion (1.2%) was rather overestimated. The number of putative HGT genes (234) in our assembly is in the range of those in nematodes (129–241) estimated with the same criterion [39] and we therefore concluded that R. varieornatus contains only a moderate number of HGT genes. Extensive HGT is thus not a common feature in the phylum Tardigrada and is also not correlated with extremotolerance, because R. varieornatus has superior tolerability compared with H. dujardini without extensive HGT. As desiccation causes severe oxidative stress [18] , desiccation-tolerant animals should have the ability to mitigate this type of stress. Multiple gene repertoire traits in the tardigrade genome suggested enhanced tolerability against oxidative stress, such as characteristic expansion of antioxidative enzymes, SODs and acquisition of bacterial-origin catalases (clade II). Bacterial clade II catalases exhibit greater resistance to denaturing conditions, such as high temperature or 7 M urea than metazoan clade III catalases [40] and, thus, tardigrade clade II catalase might be active even in hyperosmotic conditions during dehydration/rehydration and contribute to desiccation tolerance. Loss of peroxisomal oxidative enzymes including those in β-oxidation could be another strategy to adapt to oxidative stress. In peroxisomal β-oxidation, acyl-CoA oxidases catalyse the initial conversion of acyl-CoA and produce hydrogen peroxide as a side product. On the other hand, in mitochondria, similar conversion is catalysed by acyl-CoA dehydrogenases, which produce FADH 2 instead of hydrogen peroxide ( Supplementary Fig. 7 ). Thus, the lack of peroxisomal β-oxidation pathway probably leads to decreased hydrogen peroxide production during fatty acid metabolism. Decreased production of hydrogen peroxide would help the animal by preserving antioxidant capacity to combat oxidative stress during desiccation. Hydrogen peroxide produced in metazoan peroxisomes is normally decomposed by the resident enzyme, catalase. The putative decrease of hydrogen peroxide is consistent with the loss of typical metazoan catalases (clade III) in the tardigrade genome. Although the stress-responsive pathway is widely used to adapt to various environmental stresses, the decoded tardigrade genome is unexpectedly missing signalling pathways that mediate stress stimuli to inactivate mTORC1, probably leading to degradation of damaged cellular components by autophagy [41] . We speculate that the tardigrade avoids excessive destruction of cellular components after severe stress by suppressing autophagy induction and this might be beneficial to resume cellular activity by using partially damaged biomolecules after rehydration. These findings suggest that the tardigrade is insensitive to environmental stress, at least with respect to autophagy induction. Minor changes in gene expression profiles during dehydration and rehydration suggested constitutive expression of tolerance-related genes in R. varieornatus . Some tardigrade-unique genes, including putative protective proteins CAHS and SAHS, were abundantly and constitutively expressed, and could be candidates involved in desiccation tolerance. Dsup protein is a prominent example of tardigrade-unique abundant proteins involved in tolerability and is, to our knowledge, the first DNA-associating protein demonstrated to protect DNA and improve the radiotolerance of cultured animal cells. Although Dsup improved radiotolerance of HEK293 cells, cultured cell lines including HEK293 cells are potentially pre-adapted to oxidative environments in an artificial culture system and Dsup might enhance radiotolerance in conjunction with the partial adaptation of cultured cell lines. We detected ∼ 40 foci of γ-H2AX, a relatively high number, in HEK 293 cells at 1 h after 1 Gy irradiation on glass coverslips. Glass materials are reported to enhance irradiation effects approximately twofold by generating the secondary electrons [42] . Taking this effect into account, the detected number of γ-H2AX in our assay is in good accordance with previous reports in which 20 ∼ 30 DSBs were detected after 1 Gy irradiation [43] , [44] . In our comet assays, Dsup-expressing cells were irradiated on ice or treated with hydrogen peroxide at 4 °C and immediately subjected to electrophoresis, suggesting that DNA fragmentation was detected before significant DNA repair. In the γ-H2AX foci assay as well, we detected γ-H2AX foci at 1 h after irradiation when enough γ-H2AX has accumulated to be detected in human cells and the accumulation of γ-H2AX is normally retained for at least several hours [35] , [45] . Thus, we concluded that the reduced number of DNA breaks in Dsup-expressing cells was due to the suppression of DNA breaks, rather than facilitation of DNA repair processes, which is proposed in some other radiotolerant animals, such as the sleeping chironomid or rotifers [46] , [47] ( Supplementary Fig. 21 ). In some desiccation-tolerant animals, protective molecules, such as trehalose, are thought to play important roles in the protection of biomolecules against dehydration stress. Dsup could be a DNA-targeted protectant in the tardigrade, although this finding would not exclude the possibility of the presence of an effective DNA repair system, for example, expanded MRE11s could contribute to facilitation of DNA repair. Although association of proteins with DNA is potentially beneficial to physically shield DNA from environmental stress, including ROS, it could interfere with DNA replication and transcription. Indeed, overexpression of several DNA-binding proteins, such as a bacterial histone-like nucleoid-structuring protein or a small acid-soluble spore protein associated with spore DNA of Bacillus subtilis , causes severe condensation of DNA and loss of cell viability [48] , [49] . The C-terminal region of Dsup alone similarly induced an abnormal aggregation of DNA and we were unable to establish stably expressing cell lines, likely to be due to cytotoxic effects. The apparent lack of such negative effects in full-length Dsup-expressing cells suggests that the amino-terminal and middle regions play important roles to relieve the adverse effects induced by association of Dsup-C to DNA (for example, possible heterochromatinization and/or interference on transcription and replication). Dsup protein affords DNA protection without impairing cell viability and is quite suitable for future application to confer the tolerance to other animal cells. Improvement of radiotolerance by Dsup suggests that unique proteins in the tardigrades confer exceptional tolerance to harsh environmental stresses. Dsup-expressing human cultured cells exhibited better tolerance to 4 Gy of X-ray irradiation, whereas R. varieornatus exhibited far superior tolerance against high-dose irradiation, such as 4,000 Gy of He-ion beam in adults, and a lower, but still significant, dose of irradiation in mitotically active embryos (LD 50 ∼ 500 Gy) [50] . There may be additional factors besides Dsup in the tardigrade genome that contribute to the exceptional tolerance. The genome sequence and gene repertoire of the extremotolerant tardigrade revealed in this study provide a treasury of genes to improve or augment the tolerant ability in stress-sensitive animal cells. Experimental animals The YOKOZUNA-1 strain of the extremotolerant tardigrade R. varieornatus was used for all experiments. The strain was established from a single individual [4] to minimize genetic variance. The tardigrades were reared on water-layered agar plates by feeding them alga, Chlorella vulgaris (Chlorella Industry, Japan), at 22 °C [4] with additional hygienic treatment using hypochlorite. Genome size determination The genome size of the animal was determined by flow cytometry [51] . Briefly, ∼ 100 starved adult tardigrades were collected and homogenized in Galbraith buffer (pH 7.2) [52] using a Kontes Dounce tissue grinder. Dissociated cells were obtained by filtration through a CellTrics disposable filter (30 μm pore size; Partec) and stained with 50 μg ml −1 propidium iodide. The DNA content in each cell was analysed using a FACSCanto flow cytometer and FACSDiva software (BD Biosciences). The genome size was also estimated by Feulgen densitometry method [53] . Adult tardigrades were squashed on a slide glass. After air drying and fixation, the slide was hydrolysed in 5.0 N HCl and stained using Schiff reagent. The density of Feulgen stain was measured using image analysis software, FMBIO Analysis (Hitachi Software, Tokyo, Japan). In total, 119 cells from 10 animals were examined. Drosophila melanogaster was used as a reference. Genome DNA extraction After 2 days starvation and antibiotics treatment, tardigrades were extensively cleansed and genomic DNA was extracted using a Blood and Cell Culture DNA Mini Kit (Qiagen) according to the manufacturer’s protocol. Eluted DNA solution was supplemented with DNA carrier, Ethachinmate (Nippon Gene) and precipitated by ethanol. In total, ∼ 15,000 individuals were subjected to genomic analyses including whole genome shotgun (WGS), fosmid and Illumina sequencing. Fosmid library construction and sequencing The fosmid library (GRVF) was constructed from sheared genomic DNA and pKS300 cloning vector. After in vitro packaging using Gigapack III Gold Packaging Extract (Agilent Technology), the phage particles were transfected to Escherichia coli XL1-BLUE. Fosmid clone DNA from each 96-well plate was prepared by the standard alkaline lysis method (Kurabo PI-1100). End sequencing of 30,336 fosmid clones was performed using a BigDye terminator kit version 3 and the ABI 3730xl DNA Analyzers (Applied Biosystems). WGS sequencing and assembly The genome sequence of R. varieornatus was determined by using a combination of the Sanger and Illumina technologies. First, a WGS library with an average insert size of 3.5 kb was constructed. End sequencing of 489,216 clones was then performed using the ABI 3730xl DNA Analyzers (Applied Biosystems). After quality and vector clipping, the WGS and fosmid end sequence data were assembled by the PCAP.REP assembler (version 06/07/05). Gap closing and re-sequencing of low-quality regions were performed by a combination of primer walking and direct sequencing of fosmid/WGS clones and PCR products. Complete sequences of four fosmid clones were generated by the shotgun sequencing method. Second, Illumina-sequencing libraries were prepared using a Paired End DNA Sample Prep kit and a Mate Pair Library Prep kit. Paired-end (240 and 480 bp) and mate-pair (4.8, 5.8 and 7.3 kb) libraries run on the Genome Analyzer IIx sequencers (Illumina). After the pre-processing steps, de novo assembly was performed using the SOAPdenovo version 1.3. The contig sequences (8,086 contigs, total bases: 49,160,052 bp) were then incorporated into the Sanger-based assembly sequence, to close the gaps and resolve the problematic regions. RNA sequencing After 2 days starvation, extensively washed tardigrades were used. Dehydrated tardigrades were obtained by exposing the washed tardigrades to 33.8% relative humidity on a nylon mesh and filter paper. Rehydrated tardigrades were collected at 80 min and 3 h after rehydration. Total RNA was extracted using TRIzol reagent (Invitrogen). Embryos were collected at 2-day intervals after egg laying as 0–2 days and 3–4 days, and extensively washed. Six sequencing libraries were constructed from four adult samples during anhydrobiosis (hydrated, dehydrated and rehydrated at 80 min and 3 h) and two embryonic samples using a mRNA-Seq Sample Prep kit (Illumina). The sequencing was performed using the Genome Analyzer IIx and HiSeq2000 sequencers (Illumina). Full-length cDNA library construction and EST sequencing Total RNA was extracted from dehydrated tardigrades using TRIzol reagents and a full-length cDNA library (cYOK) was constructed by the oligo-capping method [54] . DNA template for each clone was amplified from the bacterial culture in a glycerol stock 384-well plate using a TempliPhi DNA amplification kit (GE Healthcare). EST sequencing of 38,400 cDNA clones was performed using the ABI 3730xl capillary sequencers (Applied Biosystems). Prediction of protein-coding genes For ab initio prediction of protein-coding genes, primary training data were created by: (1) predicting the longest open reading frames (ORFs) longer than 300 bp from the cDNA sequences; (2) screening translated ORF sequences with BLASTP [55] e -value< e −50 match against UniRef90 (ref. 56 ); (3) mapping the screened translated ORF sequences against the genome sequence using exonerate programme [57] . Thus, using the derived training data, genes were predicted from the genome sequence using SNAP [58] for initial bootstrap learning. Using the gene prediction of SNAP in the longest seven scaffolds, gene model is further trained and the final predictions were made using GlimmerHMM [59] . In parallel, RNA-seq reads were mapped to the genome sequence using TopHat software [60] and gene model was generated using cufflinks [61] . To dissociate artificial fusions of adjacent coding sequences, non-overlapping ORFs were extracted. The transcriptome-based gene model was merged with the ab initio gene model to produce the comprehensive gene set. Annotation of genes For non-coding RNAs, transfer RNAs were predicted using the combination of Aragorn v.1.2.28 (ref. 62 ) and tRNAscan-SE 1.23 (ref. 63 ), and rRNAs were predicted using RNAmmer v.1.2 (ref. 64 ). For functional annotation of protein-coding genes, sequence similarities were searched in Swiss-Prot knowledgebase [56] using BLASTP [55] with e -value< e −25, domains were searched in Conserved Domains Database [65] using RPS-BLAST with e -value< e −5 and orthologous groups were searched using KEGG Automatic Annotation Server [66] with bidirectional best hit method. Gene Ontology terms were obtained from the best Swiss-Prot match. Gene expansion and lost pathway analysis Putative orthologues in other metazoans were assigned for all tardigrade proteins based on a reciprocal BLAST search to reference protein sequences obtained from the UniProt proteome database [56] . Gene numbers were compared between the tardigrade and other metazoans. For detection of lost pathways, we assigned KEGG orthology identifiers to all tardigrade proteins and two well-established model invertebrates ( D. melanogaster and Caenorhabditis elegans ) using the KEGG Automatic Annotation Server programme [66] . We took the proteins conserved in both model invertebrates as a background and evaluated the statistical significance of missing genes in the tardigrade genome for each KEGG pathway using the KOBAS programme [67] . To find lost gene networks in addition to curated KEGG pathways, putative lost genes were inter-connected using the STRING database (cutoff score 0.9) [23] . The gene networks containing high number of putative lost genes were inspected manually. Assessment of taxonomic origin of predicted proteins BLASTP search was performed to retrieve similar proteins from the National Centre for Biotechnology Information non-redundant database for each tardigrade protein and the taxonomy information was retrieved based on their GeneInfo Identifiers. Tardigrade proteins were excluded from the retrieved list. When no similar proteins were retrieved with the defined threshold, the query proteins were classified as ‘no similarity’ ( E -value>10 −3 ) or ‘low similarity’ ( E -value>10 −5 ). The proteins exhibiting the best score with metazoan proteins were classified as ‘metazoan origin’. For rest proteins, HGT indices were calculated to assess possible foreign origin, by subtracting the bit score of the best metazoan hit from that of the best non-metazoan hit as defined previously [17] . We allowed metazoan hits with an E -value threshold of 10. The proteins with high HGT index (≥30) were classified as ‘putative HGT proteins’. The threshold value was determined as 30 in the previous work [17] . Those with a lower HGT index were classified as ‘Indeterminate’. Protein identification Chromatin fraction was separated by partial disruption and differential centrifugation [68] . Five hundred tardigrades were homogenized with a Dounce tissue grinder (Radnoti, RD440910; with 30–40 μm clearance) on ice in Buffer A (10 mM HEPES-HCl pH 7.9, 10 mM KCl, 1.5 mM MgCl 2 , 0.34 M sucrose, 10% glycerol, 1 mM dithiothreitol and Complete EDTA-free protease inhibitor cocktail (Roche)). To solubilize the cell membrane, Triton X-100 (Wako) was added to final 0.1% and incubated for 8 min on ice. The nuclear fraction was precipitated by low-speed centrifugation (4 min, 1,300 g , 4 °C) and washed twice with buffer A. The nuclear fraction was lysed by hypotonic shock in Buffer B (3 mM EDTA, 0.2 mM EGTA, 1 mM dithiothreitol and Complete EDTA-free protease inhibitor cocktail (Roche)) for 30 min on ice. After centrifugation (4 min, 1,700 g , 4 °C), insoluble chromatin was obtained as a precipitate and the supernatant was recovered as the nuclear soluble fraction. The chromatin fraction was washed two more times with Buffer B. Each fraction was analysed by SDS–PAGE and proteins were visualized using a Silver Quest Staining Kit (Invitrogen). Selective bands (B1 and B2) were excised and treated with trypsin. The fragmented peptides were analysed by nano liquid chromatography–electrospray ionization–quadrupole time of flight–tandem mass spectrometry. Proteins were identified using MASCOT software (Matrix Science; P <0.01; Mascot score cutoff was 37). Detected peptides are shown in Supplementary Table 5 . Subcellular localization analysis of GFP fusion protein For expression of GFP-fused full-length Dsup protein, the coding sequence of Dsup was amplified and inserted into Asp718 and BamHI sites of pAcGFP1-N1 (Clontech). HEK293T cells were transiently transfected with the expression construct using X-tremeGENE 9 reagent (Roche). After 24 h, the cells were stained with Hoechst 33342 (Lonza) to visualize nuclear DNA. Fluorescent signals were observed under a confocal microscope (LSM710, Carl Zeiss). Immunohistochemistry Anti-Dsup antibody was raised and affinity-purified against bacterially expressed Dsup protein. For immunohistochemistry on frozen sections, tardigrade embryos within 3 days after egg-laying were fixed with 4% paraformaldehyde at room temperature (RT) for 15 min and were embedded in Agarose-LGT (Nacalai Tesque) [32] . The embedded gels were incubated in sucrose series, 15 and 30% overnight each at 4 °C and embedded in O.C.T. Compound (Sakura Finetek Japan). Cryosections (10–14 μm thickness) were prepared using a cryostat (Leica CM1850, Leica). After three washes with 0.1% Tween 20 in Tris-buffered saline, the sections were blocked with 2% goat serum for 1 h and reacted with the affinity-purified anti-Dsup antibody (at 1/200 dilution) overnight at 4 °C and then with Alexa Fluor 488 anti-Rabbit IgG (Molecular Probes, A-11008, at 1/1,000 dilution) for 45 min at RT. Nuclear DNA was counterstained with 4′,6-diamidino-2-phenylindole (Invitrogen). Fluorescent signals were observed using a confocal microscope (LSM710, Carl Zeiss). In silico analysis based on the Dsup protein sequence Secondary structures were predicted by the CLC main workbench 6.9.1 (CLC Bio). The nuclear localization signal was predicted using the cNLS Mapper ( http://nls-mapper.iab.keio.ac.jp/ ). A hydrophobicity plot was generated by ProtScale ( http://web.expasy.org/protscale/ ) with the Kyte and Doolittle model [69] . A protein charge plot was generated using EMBOSS [70] . Subcellular localizations were predicted by WoLF PSORT [71] and TargetP [72] . DNA electrophoretic mobility shift assay The protein–DNA association was examined by a gel-shift assay [73] . Recombinant Dsup protein was produced as follows. The coding sequence of Dsup was amplified and inserted into NdeI and XbaI sites of pCold-I vector (TaKaRa), which contains the 6xHis tag at the N terminus. The construct was transformed to BL21 (DE3) cells and protein production was induced with isopropyl β- D -1-thiogalactopyranoside and cold treatment according to the manufacturer’s protocol. Recombinant Dsup protein was purified with Ni-NTA His-Bind Superflow (Novagen) in denaturing conditions using 8 M Urea and dialysed in PBS using a Micro-Dialyzer (Nippon Genetics). PBS was prepared from ten times concentrated stock solution (Wako, 163-25265). As a DNA probe, pBluescript II plasmid DNA was linearized by digestion with HindIII and subjected to the assay. Purified recombinant Dsup proteins (10, 50, 75 or 100 ng) were incubated with purified linearized pBluescript DNA (10 ng) in PBS for 20 min at RT. Purified histone H1 protein (bovine) was purchased from Upstate and was used as a positive control. After the incubation, the samples were mixed with gel loading dye (10 mM Tris-HCl pH 8.0, 1 mg ml −1 bromophenol blue, 20% glycerol) and were electrophoresed in a 0.5% agarose gel in Tris-borate-EDTA (TBE) buffer. DNA was stained with SYBR Green I and visualized by a transilluminator (ATTO). Cell lines We obtained HEK293 cells (RCB1637) and HEK293T cells (RCB2202) from RIKEN BioResource Center (BRC). The identity of these cell lines was validated by short tandem repeat profiling and all cell lines were negative for mycoplasma contamination (RIKEN BRC). The cells were maintained in Dulbecco’s modified essential medium (Nacalai Tesque) containing 10% fetal bovine serum (Corning). A Dsup expression vector was constructed by inserting the coding sequence of Dsup into KpnI and NotI sites of pCXN2KS, a modified pCAGGS vector [74] . The expression construct was transfected to HEK293 cells using X-tremeGENE 9 DNA Transfection Reagent (Roche) and stably transfected cells were selected by 700 μg ml −1 G418 (Calbiochem) treatment for 3 weeks. We observed many cells with an abnormal morphology (for example, giant cells or elongated form) and those cells could not be maintained. Clonal cell populations were obtained by limiting dilution and Dsup expression was examined by western blotting analysis and immunohistochemistry. Clones showing non-nuclear localization of Dsup protein immunoreactivity were discarded. The clone expressing the highest level of Dsup protein with nuclear localization was chosen. The target sequence for the shRNA was designed based on the online analysis software siDirect [75] and BLOCK-iT RNAi Designer ( http://rnaidesigner.lifetechnologies.com/rnaiexpress/ ) as 5′-GAA CGT AAC CGT TAC CAA AGG-3′. To construct a vector expressing shRNA, oligonucleotides encoding the stem-loop shRNA sequence were synthesized and inserted into the AgeI-EcoRI site of pLKO.1 puro [76] : the inserted sequence was 5′-ACC GGT GAA CGT AAC CGT TAC CAA AGG TTC AAG AGA CCT TTG GTA ACG GTT ACG TTC TTT TTG AAT TC-3′. The shRNA expression construct was transfected to the Dsup-expressing stable cell line. After selection by 2 μg ml −1 puromycin (Sigma) treatment, cell cloning was performed as described above. Comet assay A comet assay was performed using the CometAssay Kit (Trevigen) under alkaline or neutral conditions essentially according to the manufacturer’s protocol. Briefly, cells were irradiated on ice using an X-ray generator, the Pantak HF 350 (Shimadzu) operating at 200 kV–20 mA with a filter of 0.5 mm Cu and 1 mm Al at a fixed dose rate of 1.73 Gy min −1 . We selected irradiation doses that increased the proportion of tail DNA to a 30–50% of total DNA to clearly visualize the irradiation-dependent increase of DNA damage without catastrophic fragmentation (10 and 5 Gy were used for alkaline or neutral conditions, respectively). The irradiated cells were immediately trypsinized and collected as a cell suspension. Cell suspensions were mixed with molten agarose and solidified as a thin layer on slide glasses by chilling at 4 °C for 30 min. For alkaline comet assays, the slide glasses were soaked for 1 h in manufacturer’s lysis solution (Trevigen) at 4 °C for 1 h to lyse the cells and then immersed in alkaline solution (200 mM NaOH, 1 mM EDTA pH>13) for 1 h at RT, in the dark and electrophoresed in freshly prepared alkaline solution at 25 V and 4 °C for 1 h. For neutral comet assay, the cell-mounted slide glasses were soaked in the lysis solution (2.5 M NaCl, 10 mM Tris, 100 mM EDTA, 1% sarcosinate and 0.01% Triton X-100) at 4 °C [77] and then washed in TBE buffer for 30 min and electrophoresed in freshly prepared TBE buffer at 25 V and 4 °C for 1 h. After electrophoresis, the comets were visualized by staining with SYBR Green I and captured with an Imager Z1 (Carl Zeiss). DNA fragmentation was quantified for at least 120 comets per condition using CASP software [78] . Hydrogen peroxide treatment Cells were treated with 100 μM hydrogen peroxide (H 2 O 2 ) at 4 °C for 30 min. Half of the cells were pretreated with an antioxidant, 10 mM NAC (Sigma) for 30 min before the hydrogen peroxide treatment. DNA damage was evaluated by the alkaline comet assay with the electrophoresis at 25 V at 4 °C for 30 min, immediately after the treatment. At least 302 comets were analysed for each condition. γH2AX foci detection The cultured cells on Chambered Coverglass (Thermo Scientific) were irradiated with 1 Gy of X-ray using the Pantak HF 350 X-ray generator (Shimadzu). One hour after X-ray irradiation, the cultured cells were fixed with 4% formaldehyde for 15 min and permeabilized with 0.5% Triton X-100 for 15 min. The cells were blocked with 10% goat serum for 1 h and reacted with the anti-phospho-histone H2A.X (Ser139) antibody clone JBW301 (Merck Millipore, 05-636, at 1/800 dilution) for 1 h and then with Alexa Fluor 488 anti-mouse IgG (Molecular Probes, A-11001, at 1/500 dilution) for 45 min. Nuclear DNA was counterstained with 4′,6-diamidino-2-phenylindole (Invitrogen). All reactions and procedures were essentially performed at RT. Fluorescent signals were observed by confocal microscopy (LSM710, Carl Zeiss). The depth-coded projections were captured as stacks of ten optical sections of z-series at 1-μm intervals and converted to binarized images by ImageJ version 1.47. The threshold value for image conversion was manually adjusted until a visual best fit between the original and converted images was observed ( Supplementary Fig. 22 ). The numbers of γ-H2AX foci were counted using the ImageJ software [79] . Quantification of Dsup transcript by realtime reverse transcriptase–PCR Total RNA was extracted from cell pellet using the RNeasy mini kit following the manufacturer’s instructions (Qiagen) and reverse-transcribed using PrimeScript RT reagent Kit with gDNA Eraser (Perfect Real Time; TaKaRa). Dsup expression was quantified by real-time PCR using LightCycler 480 Instrument II (Roche) and knockdown efficiency was calculated. Human β-actin was used as an internal control. Sequences for primer sets were as follows: Dsup : forward 5′-TCC ACA GAA CCC TCT TCC AC-3′ and reverse 5′-TCT TGA CAA TGG CAG CTG AG-3′. β-actin : forward 5′-TGA GCG CGG CTA CAG CT-3′ and reverse 5′-TCC TTA ATG TCA CGC ACG ATT T-3′. Cell cycle analysis Cell cycle analysis was performed using flow cytometry based on DNA content and incorporation of 5-bromo-2-deoxyuridine (BrdU) [80] . BrdU (Sigma) was added to cell cultures at 10 μM at 37 °C for 1 h. After pulse labelling, the cells were collected as a cell suspension by trypsinization. Cells were fixed with 90% ice-cold ethanol with gentle vortexing and incubated on ice for 1 h. Cells were rinsed in PBS and further incubated with 2 N HCl/0.5% Triton X-100 at RT for 30 min. After that, cells were suspended in 0.1 M sodium tetraborate for 30 min. Cells were incubated with 1/50 diluted anti-BrdU mouse IgG (555627, BD Pharmingen) at RT for 1 h and reacted with 1/500 diluted Alexa Fluor 488 anti-mouse IgG (Molecular Probes, A-11001) for 30 min after two washes with PBS. Cells were finally incubated with PBS containing 10 μg ml −1 RNase (Sigma) and 5 μg ml −1 propidium iodide (Dojindo) at RT for 30 min in the dark and then filtered through 77-μm nylon mesh to remove cell clusters. Cells were analysed by flow cytometry using BD FACSVerse (BD Bioscience). At least 10,000 events were collected and data were analysed using FlowJo software (Tree Star Inc.). Cell count and measurement of cell viability Cells were seeded in poly- L -lysine-coated 24-well plates (Iwaki) at a density of 1,000 cells per well. After 24-h incubation (1 dps), the cells were irradiated with 4 Gy of X-ray using the Pantak HF 350 X-ray generator. With 24 h intervals, the cells were incubated with PrestoBlue Cell Viability Reagent (Invitrogen) for 2 h and the fluorescence was measured using a microplate fluorometer, the Spectra max Gemini EM (Molecular Devices). To count the cell number, the cells were washed gently with PBS and treated with trypsin, then recovered as a cell suspension at 8, 10 and 12 dps. The numbers of cells in the suspensions were counted using an automatic cell counter, the Z1 Particle Counter (Beckman Coulter). We examined three wells for each condition. Statistical analysis The effects of Dsup or its derivatives in alkaline/neutral comet assays, γ-H2AX assays and cell viability assays were evaluated by statistical tests. For pairwise comparisons, two-tailed Student’s t -test or two-tailed Welch’s t -test was used depending on the equality of variance between samples determined by F-test (significance level=0.05). For comparisons among three or more samples, Tukey–Kramer’s test was used to evaluate the differences between all possible comparison pairs. All statistical measures and tests of the comet assays, γ-H2AX assays and cell viability assays are provided in Supplementary Tables 6–15 . Data availability All sequence data were deposited to DDBJ/GenBank/EMBL under the accession numbers: (i) BDGG01000001–BDGG01000199 for the nuclear genome scaffolds, (ii) AP017609 for the assembled mitochondrial genome, (iii) FT955276–FT997721 for the GRVF end sequences, (iv) AP013349–AP013352 for the complete sequences of fosmid clones, (v) HY377478–HY448296 for the EST sequences of full-length cDNA clones and (vi) 2343876328–2344039843, 2343537664–2343876048 and 2343264041–2343530383 for WGS trace data. All Illumina sequence reads were deposited to the DDBJ Sequence Read Archive (DRA) under accession numbers (i) DRA001119 for WGS and (ii) DRA001120 for RNA-seq. The sequence of Dsup has been submitted to DDBJ with the accession number, LC050827. The corresponding Bioprojects were deposited to DDBJ/GenBank/EMBL under the accession numbers: PRJDB5011 (Umbrella), PRJDB4588 (Genome assembly), PRJDB1451 (genome short reads), PRJDB2359 and PRJDB2360 (RNA-seq data). The genome browser and the relevant databases are available at http://kumamushi.org/ . How to cite this article: Hashimoto, T. et al . Extremotolerant tardigrade genome and improved radiotolerance of human cultured cells by tardigrade-unique protein. Nat. Commun. 7:12808 doi: 10.1038/ncomms12808 (2016).